Small GTPase Rab37 targets tissue inhibitor of metalloproteinase 1 for exocytosis and thus suppresses tumour metastasis Rab small GTPases are master regulators of membrane trafficking and guide vesicle targeting. Recent publications show that Rab-controlled trafficking pathways are altered during tumorigenesis. However, whether any of the Rabs plays a metastasis suppressor role is least explored. Here we address the metastasis suppressive function of human Rab37 (hRAB37) using secretomics, cell, animal and clinical analyses. We show that tissue inhibitor of metalloproteinase 1 (TIMP1), a secreted glycoprotein that inhibits extracellular matrix turnover, is a novel cargo of hRAB37. hRAB37 regulates the exocytosis of TIMP1 in a nucleotide-dependent manner to inactivate matrix metalloproteinase 9 (MMP9) migration axis in vitro and in vivo . Dysfunction of hRAB37 or TIMP1 abrogates metastasis suppression. Lung cancer patients with metastasis and poor survival show low hRAB37 protein expression coinciding with low TIMP1 in tumours. Our findings identify hRAB37 as a novel metastasis suppressor Rab that functions through the TIMP1-MMP9 pathway and has significant prognostic power. Rab proteins are members of the Ras superfamily of GTPases that switch between GDP-bound (inactive) and GTP-bound (active) forms. They transport cargo proteins to target membrane, organelle and cellular compartment to coordinate the cell membrane dynamics, cytoskeleton organization, signal transduction and membrane trafficking [1] , [2] . Recent publications show that Rab-controlled trafficking pathways are altered during tumour development and progression. Overexpression of Rab8, Rab11, Rab21, Rab23, Rab25 and Rab27B (refs 3 , 4 , 5 , 6 , 7 , 8 , 9 ) promotes cancer cell migration and tumour invasion. For example, oncogenic Rab8 transports exocytic vesicles carrying MT1-matrix metalloproteinase (MMP) to the matrix degradation sites at the plasma membrane (PM) of migrating cancer cells cultured in collagen gel [3] . An increased expression of Rab27B is associated with the poor prognosis of oestrogen receptor-positive breast cancer patients. Through mass spectrometric (MS) analysis, heat-shock protein 90α has been identified as a component of Rab27B-regulated vesicles and it acts as a pro-invasive growth regulator required for MMP2 activation [6] . Previous studies indicate that Rab25 functions as a tumour suppressor or oncogene depending on the cancer type [10] , [11] , [12] . In addition, loss of Rab21 correlates with increased malignancy in prostate and ovarian cancer [13] . Although there are >60 members in the Rab family, whether any of the Rabs plays a role in metastasis suppression is least explored. We previously cloned the human Rab37 ( hRAB37 ) residing in chromosome 17q25 (accession number NM_001006638) and demonstrated that hRAB37 was downregulated mainly by promoter hypermethylation in lung cancer cells and patients, and low mRNA expression of hRAB37 gene was associated with tumour metastasis in lung cancer patients [14] . We speculated that the hRAB37 may act as a metastasis suppressor in lung cancer. The murine Rab37 (mRab37) was found in secretory granules of bone marrow mast cell [15] . Rab37 together with Rab3, Rab26, Rab27A and Rab27B are referred to as secretory Rabs owing to their localization in secretory granules [1] . Therefore, hRAB37 may function as a regulator in exocytotic pathway. Notably, mRab37 co-localizes with TNF-α-containing vesicles in activated macrophages [16] . In addition, mRab37 is involved in the control of insulin exocytosis in murine pancreatic β-cells [17] , [18] . However, more investigation is required to identify the cargos of hRAB37 and to dissect the defect mechanism of hRAB37 in human disease such as cancer. Here we undertook several evidence-based studies to answer our four main questions. Is hRAB37 involved in transportation of exocytotic vesicles or recycling vesicles? What consequences can hRAB37 alteration have on cell migration and metastasis? Are any of the trafficking cargos important for hRAB37-mediated motility control? If so, what are the underlying mechanisms of metastasis suppression by hRAB37 and its cargo? Tissue inhibitor of metalloproteinase 1 (TIMP1) is a secreted protein that inhibits MMPs and extracellular matrix turnover thereby decreasing cell motility [19] , [20] , [21] but very little is known [22] about its mode of secretion. Our results provide first compelling evidence from lung cell, animal and clinical studies that hRAB37 is a metastasis suppressor. It suppresses metastasis through regulating TIMP1 for exocytosis to extracellular compartment leading to inactivation of MMP9 invasion signalling. The results of the present study have clinical implication for cancer prognosis prediction. hRAB37 is involved in transportation of exocytotic vesicles Secretory pathways include tranportation of secretory granules and endocytic recycling vesicles [1] , [2] . To dissect the trafficking pathway regulated by hRAB37 protein, we first compared the cellular distribution of endogenous hRAB37 with several organelle markers in CL1-0 lung cancer cell with low motility and high endogenous hRAB37 (ref. 14 ) using immunofluorescence confocal analyses. The markers included secretory granule marker VAMP2 and early endosome marker EEA1. Merged confocal images demonstrated the co-localization of endogenous hRAB37 with VAMP2, but not with endosome marker EEA1 ( Fig. 1a ). Ectopically expressed wild-type (WT) hRAB37 protein in CL1-5, an isogenic cell line derived from CL1-0 with high motility and low hRAB37 (ref. 14 ), showed cellular distributions similar to endogenous hRAB37 ( Fig. 1b ) where it co-localized more with secretory granule marker than with endosome marker. Figure 1: hRAB37 mediates trafficking of exocytotic vesicles and not recycling vesicles. ( a , b ) Representative images of double immunofluorescence analysis of endogenous hRAB37 (red) in CL1-0 cells ( a ) and ectopically expressed Flag-hRAB37 (red) in CL1-5 cells ( b ), and cellular compartment markers (green) including secretory granule marker VAMP2 and early endosome marker EEA1. Enlarged images shown in insets of the merged panel. hRAB37 co-localized more with VAMP2 than with EEA1. Scale bars, 10 μm. ( c ) Epifluorescence microscopy images of VSVG transport in control and Rab37KD COS1 cells transfected with VSVG-ts-GFP. Cells were fixed at indicated time points after releasing from temperature block and stained by 4',6-diamidino-2-phenylindole (DAPI, blue). Transport of VSVG-ts-GFP to the PM was impaired by Rab37KD. VSVG signals were mainly retained in the perinuclear region and intracellular vesicles (comparing the 120-min images in control and Rab37KD groups). ( d ) Quantification of cells displaying VSVG-GFP on the PM at 60 and 120 min among cells transfected with control or Rab37KD oligos. Each measurement was from an average of 150 transfected cells. Data are mean±s.e.m. ( n =3). P values determined using two-tailed Student’s t -test. ( e ) Quantification of intracellular AlexaFluor488-Tfn in control and Rab37KD COS1 cells by ELISA assay. The relative amount of residual intracellular AlexaFluor488-Tfn compared with time point zero was calculated. Data are mean±s.e.m. ( n =3). ( f ) Immunoblots of Rab37 expression in control and Rab37KD COS1 cells. Normalized fold changes were analysed and labelled below the blots. Full size image We further performed quantitative analyses of vesicular stomatitis virus ts045 G protein fused to green fluorescent protein (VSVG-ts-GFP) exocytosis from endoplasmic reticulum through the Golgi to the PM [22] , [23] in Rab37 knockdown (Rab37KD) or control COS1 cells ( Fig. 1c ). As shown in epifluorescence microscopy images at 15 min after shifting to a permissive temperature, the arrival of VSVG-ts-GFP to the Golgi was observed in both control and Rab37KD cells. However, the subsequent transport of VSVG-ts-GFP to the PM was impaired by Rab37KD. VSVG signals were mainly retained in the perinuclear region and intracellular vesicles (comparing the 120-min images in control and Rab37KD groups; Fig. 1c ). Quantification was performed in 150 cells transfected with control or Rab37KD oligos in three independent experiments ( Fig. 1d ). To discriminate whether hRAB37 was involved in secretion or endocytic recycling, we also performed quantitative analyses for the recycling of endocytosed transferrin receptor (TfnR) [24] , [25] ( Fig. 1e ). Of note, the recycling of internalized TfnR did not show difference between control and Rab37KD COS1 cells at any of the time points examined ( Fig. 1e ). KD efficiency was checked by immunoblotting ( Fig. 1f ). All together, these results indicated that hRAB37 is involved in the exocytotic pathway of nascent secretory protein from the Golgi to the PM but not in the recycling endosome-mediated secretory pathway. TIMP1 localizes in hRAB37-containing vesicles Thus far, the putative cargos identified for mRab37 are TNF-α in murine macrophage and insulin in murine pancreatic cell lines [16] , [18] . To identify the cargos of hRAB37, we performed an unbiased proteomics screen of conditioned medium (CM) from control and ectopically expressed hRAB37-WT CL1-5 cells. Among the 185 proteins that were identified with high confidence in two separate experiments, secreted TIMP1 level was increased in CM from WT compared with that from control ( Supplementary Data 1 and Supplementary Fig. 1 ). We focused on TIMP1 because it is a secreted glycoprotein that inhibits extracellular matrix turnover thereby decreasing cell motility, but very little is known about its mode of secretion. To validate our proteomics results, protein levels of TIMP1 and TNF-α in the CM were examined in CL1-5 cells treated with exocytosis inhibitor EXO1. hRAB37-mediated TIMP1 secretion was blocked by EXO1 in a dose-dependent manner and TNF-α secretion was also inhibited, although to a lesser extend owing to low basal secretion level in CL1-5 cells ( Supplementary Fig. 2 ). To further determine whether TIMP1 was actually present in hRAB37-containing vesicles in various cell types, we performed biochemical and microscopic analyses. We found that TIMP1 was associated with hRAB37 in the same vesicle lysate fractions using immunoprecipitation western assay ( Fig. 2a ). We then performed immunogold electron microscopy (immuno-EM) assay for ultrastructural localization of hRAB37 and TIMP1, and found that the endogenous Rab37 and TIMP1 localized on the same vesicles in COS1 cell and mouse lung tissue ( Fig. 2b ). Figure 2: hRAB37 co-localizes with TIMP1 in the same vesicular structures. ( a ) Vesicles of CL1-5 cells, expressing Flag-tagged hRAB37 protein, were isolated by two centrifugations first at low speed and then at high speed. Supernatant containing vesicles were immunoprecipitated (IP) with anti-Flag beads and lysates were blotted for Flag-tagged hRAB37 and endogenous TIMP1. More TIMP1 was associated with hRAB37-containing vesicles than with control vesicles. ( b ) Ultrastructural localization of hRAB37 and TIMP1 illustrated by immuno-EM images of COS1 cell (left) and mouse lung tissue (right). Samples were fixed, sectioned and incubated with indicated antibodies coupled to gold particles, and images were taken by EM. Rab37 (10 nm of gold, arrow) and TIMP1 (15 nm of gold, arrow head) localized to the same vesicles. Scale bars, 100 nm. ( c ) TIMP1 localizes in hRAB37-containing vesicles in a nucleotide-dependent manner. Immuno-EM images show co-localization of hRAB37 (arrow) and TIMP1 (arrow head) in control, WT (wild-type) and Q89L (the GTP-bound active mutant), but not in T43N (the GDP-bound inactive mutant) CL1-5 cells. G, Golgi. Scale bars, 100 nm. ( d ) Co-localization of both TIMP1 and hRAB37 in the same vesicle was quantified in 100 TIMP1-containing vesicles each in control, WT, Q89L and T43N cells by two independent immuno-EM experiments. Quantification of co-localization of hRAB37 and TIMP1 in 100 vesicles counted is shown as a percentage in the graph. Data are mean±s.e.m. ( n =2). P values determined using two-tailed Student’s t -test. Full size image Next, we determined whether TIMP1 localized in hRAB37-containing vesicles in a nucleotide-dependent manner. To this end, we established four stable clones in CL1-5 cells, including empty vector control (control), Flag-hRAB37-WT, Flag-hRAB37-Q89L (Q89L) constitutively active GTP-bound mutant and Flag-hRAB37-T43N (T43N) dominant-negative GDP-bound mutant cells. We measured TIMP1 and hRAB37 co-localization proportion of 100 TIMP1-containing vesicles each in control, WT, Q89L and T43N cells by immuno-EM in two independent experiments. Strikingly, WT and Q89L cells showed significantly higher co-localization proportion (WT: 46%, Q89L: 50%) than those in control cells (12%). Conversely, there was a marked reduction of co-localization proportion (13%) in T43N cells ( Fig. 2c,d ). Our quantitative immuno-EM studies also revealed that T43N-hRAB37 displayed 20% more distribution at the nuclear periphery region and lost membrane binding to the vesicles compared with WT- and Q89L-hRAB37 ( Supplementary Fig. 3 ). Collectively, these results demonstrate that TIMP1 localizes in hRAB37-containing vesicle in a nucleotide-dependent manner. TIMP1 is a trafficking cargo of hRAB37 Furthermore, we determined whether hRAB37 could mediate TIMP1 secretion in a nucleotide-dependent manner. Confocal immunofluorescence microscopy of four established stable clones of CL1-5 cells demonstrated that TIMP1 and hRAB37 co-localized in WT and Q89L cells, whereas TIMP1 and hRAB37 were distributed to distinct regions in the T43N inactive hRAB37 cells ( Fig. 3a ). Importantly, higher concentrations of TIMP1 in CM from WT and Q89L cells compared with control and T43N cells were found ( Fig. 3b ). These data indicated that hRAB37 regulates TIMP1 secretion in a nucleotide-dependent manner. Notably, although RAB8a transports exocytic vesicles, it did not regulate TIMP1 secretion ( Supplementary Fig. 4 ). These results further support the notion that hRAB37 specifically regulated TIMP1 secretion. Figure 3: hRAB37 regulates TIMP1 trafficking in a nucleotide-dependent manner. ( a ) Confocal microscopy images of hRAB37 (red), TIMP1 (green) and nucleus staining (blue) in control, WT, Q89L and T43N-hRAB37 expressed CL1-5 cells. Enlarged images shown in insets of the merge panel. Scale bars, 10 μm. hRAB37 and TIMP1 were distributed to distinct regions in the T43N GDP-bound inactive mutant cells. ( b ) Immunoblots of TIMP1 secretion level in CM showed that higher concentrations of TIMP1 in CM from WT and Q89L cells compared with control and T43N cells. ( c , d ) Selected frames from time-lapse movies of TIRF images of CL1-5 cells expressing RFP-tagged hRAB37 and GFP-tagged TIMP1 (hRAB37-RFP+TIMP1-GFP) ( c ) or cells expressing RFP and GFP vector control (Vector-RFP+Vector-GFP) ( d ). hRAB37-mediated TIMP1 trafficking was observed in cells co-expressing hRAB37 and TIMP1 as described in the text. Enlarged images of the boxed areas from time-lapse movies with time intervals in minutes and seconds are shown (bottom). Arrow indicates trafficking vesicle. Scale bars, 10 μm. ( e ) For quantification of vesicle trafficking event, we defined each yellow fluorescence spot as a TIMP1-containing vesicle trafficked by hRAB37, and then tracked each yellow vesicle trafficking distance with trackIT software. We measured the ratio between the moving yellow vesicles and the total yellow vesicles in the cell. Each measurement is an average of 20 co-localized vesicles in cell. Data are mean ±.s.e.m. ( n =6). P values were determined using two-tailed Student’s t -test. Full size image For real-time visualization of the effect of hRAB37 on TIMP1 trafficking, CL1-5 cells were analysed using two-colour total internal reflection fluorescence (TIRF) microscopy, which permits selective visualization of fluorescently labelled vesicles located in close proximity to the PM. The penetration depth of our TIRF evanescence field was measured to be ~100 nm. The TIRF images of cells co-transfected with red fluorescent protein (RFP)-tagged hRAB37 and GFP-tagged TIMP1 illustrated the co-localized yellow fluorescent vesicles, which were defined as TIMP1-containing vesicles trafficked by hRAB37. These co-localized vesicles appeared quickly and diffused laterally from the point of insertion within the PM in the TIRF evanescence field ( Fig. 3c and Supplementary Movie 1 ), while the fluorescence signals remained steady in cells co-transfected with empty vectors of RFP and GFP ( Fig. 3d , Supplementary Fig. 5 and Supplementary Movie 2 ). To obtain a quantitative measurement of vesicle trafficking event, we tracked the position of the yellow vesicles and measured the ratio between the moving yellow vesicles and the total yellow vesicles in the cell. While vesicle trafficking events were low in vector control cells, they were markedly enhanced in cells co-transfected with RFP-tagged hRAB37 and GFP-tagged TIMP1 ( Fig. 3e ). To the best of our knowledge, this is the first report on the dynamics of hRAB37-mediated trafficking and docking of TIMP1-containing vesicles to the PM. hRAB37 suppresses metastasis in a nucleotide-dependent manner We previously showed that promoter hypermethylation and low mRNA expression of hRAB37 gene correlated with increased tumour metastasis potential in lung cancer patients [14] . Therefore, we hypothesized that hRAB37 may be a metastasis suppressor. To test this hypothesis, we performed migration and invasion assays on established stable cells of control, WT, Q89L (the GTP-bound active mutant) and T43N (the GDP-bound inactive mutant) derived from CL1-5. The CL1-5 high-invasive lung cancer cell line with low expression of endogenous hRAB37 provides a good model to study hRAB37-mediated metastasis suppression. The results showed that WT and Q89L cells reduced migration and invasion abilities compared with the control and dominant-negative T43N mutant cells ( Fig. 4a,b ). To confirm that this is not unique to CL1-5 cells, we also performed invasion assays with other human lung cancer cells including A549 lung adenocarcinoma cell line and H460 large-cell lung cancer cell line. Similarly, transient overexpression of WT-hRAB37 exerted an invasion suppressive function in multiple lung cell models ( Supplementary Fig. 6 ). Figure 4: hRAB37 suppresses lung cancer invasion and tumour metastasis in a nucleotide-dependent manner in vitro and in vivo. ( a , b ) Migration ( a ) and invasion ( b ) assays in control, WT, Q89L and T43N-hRAB37 expressed CL1-5 cells. Scale bars, 100 μm. ( c ) Invasion assay of CL1-5 cells treated with CM from the control, WT, Q89L and T43N cells. TIMP1 concentrations in CM measured by ELISA assay are as indicated (bottom). ( d ) Invasion assay of control, WT, Q89L and T43N cells treated with TIMP1 recombinant protein. Scale bars, 100 μm. The transwell migration and invasion abilities were quantified and normalized to control group shown as a percentage in the graph (right). P values determined using two-tailed Student’s t -test. Data represent mean±s.e.m. ( n =4). ( e ) Immunoblots for cytosolic expression of hRAB37 and β-actin, as well as TIMP1 secretion in CM are shown. Gelatin-zymography assay for MMP9 activity are shown with pro-form and active form labelled as indicated. ( f ) Four representative lung images from BALB/c nude mice intravenously injected via tail vein with CL1-5 cells expressing control, WT, Q89L and T43N-hRAB37. ( g ) H&E stains show more lung colonization and bigger tumour mass in control and T43N inactive hRAB37 groups compared with WT and Q89L groups. Scale bars, 400 μm. Number of tumour nodules in control, WT, Q89L and T43N mice groups are shown in the graph (right). Data are mean±s.e.m. P values were calculated by two-tailed Student’s t -test ( n =8 mice per group). ( h ) Immunohistochemistry was performed on lung tissues from control, WT, Q89L and T43N mice to detect the expression level of hRAB37 and TIMP1 proteins. The concordant expression between hRAB37 and TIMP1 was confirmed except for the tumours derived from the T43N inactive hRAB37 group. Scale bars, 100 μm. Full size image We have demonstrated that hRAB37 is important in the control of TIMP1 exocytosis to CM, therefore, we proposed that hRAB37 functions in the context of TIMP1 exocytosis to regulate cancer motility. To verify this, we first treated highly metastatic CL1-5 cells with CM from cells expressing control, WT, Q89L and T43N, and then performed invasion assays. Inhibition of invasion was observed by treatment of CL1-5 cells with CM collected from WT and Q89L expressed cells but not T43N inactive hRAB37 cells ( Fig. 4c ). Notably, the concentrations of TIMP1 measured in CM were entirely consistent with the scenario that hRAB37 transported TIMP1 to inhibit cell migration and invasion ( Fig. 4c ). Importantly, control and T43N cells, which secreted TIMP1 at low level, reduced invasion abilities by treatment with TIMP1 recombinant protein ( Fig. 4d ). TIMP1 is known to inactivate MMP9 activity [19] , [20] , [26] . Accordingly, gelatin-zymography assay revealed that MMP9 activity was inhibited in WT and Q89L cells compared with control and T43N cells ( Fig. 4e ). In addition, MMP9 activity inversely correlated with TIMP1 level in CM from the other hRAB37 reconstituted lung cancer cells ( Supplementary Fig. 6 ). Migration signalling proteins such as p-FAK and GTP-RhoA were downregulated in WT and Q89L cells compared with the control ( Supplementary Fig. 7a,b ). These data suggested that the suppression of migration and invasion by hRAB37 is mediated via TIMP1 secretion to inactivate MMP9 activity in a nucleotide-dependent manner. The strong inhibition of cell migration and invasion in cell model prompted us to determine whether hRAB37 acted as a tumour metastasis suppressor in animals. Control, WT, Q89L and T43N cells were tail-vein injected into BALB/c nude mice. Eight weeks post injection, the mice were killed, and their lungs were collected for analysis of tumour extravasation and colonization. We found that WT and Q89L markedly inhibited metastases to mouse lungs compared with control and T43N groups ( Fig. 4f,g ). Importantly, the concordant expression between hRAB37 and TIMP1 was confirmed in vivo except for the tumours derived from T43N inactive hRAB37 group that showed high hRAB37 expression and low TIMP1 staining ( Fig. 4h ). KD of hRAB37 promotes metastasis in vitro and in vivo Next, we undertook a KD approach to further verify that hRAB37 was a metastasis suppressor. Importantly, stable hRAB37KD H460 lung cancer cells showed increased migration and invasive potential compared with control ( Fig. 5a,b ). Note that hRAB37KD significantly reduced TIMP1 secretion in CM leading to MMP9 activation ( Fig. 5c and Supplementary Fig. 8c ). Similar results were obtained in reconstitution experiments after KD of ectopically expressed WT-hRAB37 in CL1-5 cells (WT-hRAB37KD; Supplementary Fig. 8a,b ). Migration signalling proteins such as p-FAK and GTP-RhoA were upregulated in hRAB37KD cells compared with the control ( Supplementary Fig. 7c ). Figure 5: KD of hRAB37 promotes lung cancer invasion and tumour metastasis in vitro and in vivo. ( a , b ) Migration ( a ) and invasion ( b ) assays of stable KD control (sh-Con) and two hRAB37KD clones (sh1 and sh2). Scale bars, 100 μm. The transwell migration and invasion abilities were quantified and normalized to control group shown as a percentage in the graph (right). P values determined using two-tailed Student’s t -test. Data represent mean±s.e.m. ( n =3). ( c ) Immunoblots for cytosolic expression of hRAB37 and β-actin, as well as TIMP1 secretion in CM are shown. Gelatin-zymography assay for MMP9 activity are shown. The positions of pro-form and active form of MMP9 are as indicated. ( d , e ) Stable KD control (sh-Con) and two hRAB37KD clones (sh1 and sh2) H460 cells were injected into the left lateral thorax of Balb/c nude mice. The right lateral lungs were isolated and prepared for pathological examination at 4 weeks post injection. ( d ) H&E stains show more lung colonization and bigger tumour mass in sh1 and sh2 groups compared with sh-Con group in the right lateral lung. Scale bars, 300 μm. ( e ) Number of tumour nodules and number of mice that developed metastasis in sh-Con, sh1 and sh2 groups are shown. Data are mean±s.e.m. P values were calculated by two-tailed Student’s t -test ( n =8 mice per group). ( f ) Immunohistochemistry was performed on lung tissues from sh-Con, sh1 and sh2 mice to detect the expression level of hRAB37 and TIMP1 proteins. Concordantly, low expression of hRAB37 and TIMP1 was confirmed in metastatic lung nodules of sh1 and sh2 groups as compared with sh-Con group. Scale bars, 100 μm. Full size image Lung-to-lung metastasis in animal model was performed using stable hRAB37KD H460 cells. Cancer cells were inoculated percutaneously into the left lateral thorax, and the tumour nodules at the right lungs of injected mice were determined by haematoxylin and eosin (H&E) staining. Strikingly, hRAB37KD significantly promoted lung-to-lung tumour metastases by sixfold compared with the control ( Fig. 5d,e ). Of note, concordantly low expression of hRAB37 and TIMP1 was confirmed in metastatic lung nodules in vivo ( Fig. 5f ). All these data corroborated with the hRAB37 overexpression results, indicating that hRAB37 is a bona fide metastasis suppressor. TIMP1 is essential to hRAB37-mediated metastasis suppression To further verify the role of TIMP1 in hRAB37-mediated metastasis suppression, migration and invasion assays using WT-hRAB37 (WT-Con), TIMP1KD in the WT-hRAB37 background (WT-TIMP1KD) and TIMP1 reconstitution by addition of TIMP1 recombinant protein (WT-TIMP1KD+TIMP1) were performed. WT-TIMP1KD showed an increase of cell migration and invasion, whereas WT-TIMP1KD+TIMP1 abolished the migration and invasion ability ( Fig. 6a,b ). Similar results were obtained with the TIMP1 reconstituted Q89L-hRAB37 cells ( Supplementary Fig. 9 ). Treatment of T43N cell, which secreted TIMP1 at low level, with TIMP1 recombinant protein also reduced the migration and invasion ability ( Supplementary Fig. 10a,b ). In addition, MMP9 activity inversely correlated with TIMP1 level in CM from the reconstituted cells ( Fig. 6c ). These data suggested that TIMP1 secretion to inactivate the MMP9 activity attributes to metastasis suppression by hRAB37. Figure 6: hRAB37 inhibits lung cancer metastasis in vitro and in vivo via TIMP1. ( a , b ) Migration ( a ) and invasion ( b ) assays of WT-hRAB37 (WT-Con), TIMP1KD (WT-TIMP1KD) and reconstituted TIMP1 by adding TIMP1 recombinant protein (WT-TIMP1KD+TIMP1). Scale bars, 100 μm. WT-TIMP1KD showed an increase in cell migration and invasion, whereas WT-TIMP1KD+TIMP1 abolished the migration and invasion ability. The transwell migration and invasion abilities were quantified and normalized to control group shown as a percentage in the graph (right). P values determined using two-tailed Student’s t -test. Data represent mean±s.e.m. ( n =3). ( c ) Immunoblots of TIMP1 and gelatin-zymography assay for MMP9 activity in CM are shown with pro-form and active form of MMP9 labelled as indicated. ( d ) Four representative lung images from BALB/c nude mice intravenously injected via tail vein with CL1-5 cells indicated. ( e ) H&E stains show more lung colonization and bigger tumour mass in WT-TIMP1KD group compared with WT-Con and WT-TIMP1KD+TIMP1 groups. Scale bars, 400 μm. Number of tumour nodules in WT-Con, WT-TIMP1KD and WT-TIMP1KD+TIMP1 mice groups are shown in the graph (right). Data are mean±s.e.m. P values were calculated by two-tailed Student’s t -test ( n =8 mice per group). Full size image We further investigated the interplay between hRAB37 and TIMP1 on anti-metastasis effects in animals. WT-Con, WT-TIMP1KD and WT-TIMP1KD+TIMP1 cells were tail-vein injected into BALB/c nude mice, and the mice were observed for tumour extravasation and colonization to lungs. Notably, WT-TIMP1KD mice showed more tumour nodules than WT-Con mice, while such aggressive tumour metastasis phenotype was attenuated in WT-TIMP1KD+TIMP1 mice ( Fig. 6d,e ), suggesting that the metastasis inhibition of hRAB37-WT GTPase is mediated by TIMP1. In addition, TIMP1 treatment dramatically inhibited lung cancer metastasis of the animal group tail-vein injected with high metastatic T43N cells ( Supplementary Fig. 10c,d ). Together, these data indicated that TIMP1 secretion is crucial to hRAB37-mediated tumour metastasis suppression. Clinical impacts of concordantly low hRAB37/TIMP1 expression Since hRAB37 promotes TIMP1 secretion to inhibit migration and invasion in cell model and tumour metastases in animal model, we further investigated whether low hRAB37 protein expression correlated with low TIMP1 level in cancer patients with cancer metastasis and poor prognosis. For this, we examined the expression of hRAB37 and TIMP1 in lung tumour specimens from 165 lung cancer patients by immunohistochemical analysis ( Fig. 7a ). Importantly, a total of 47.3% (78/165) patients showed low hRAB37 protein expression ( Table 1 and Supplementary Table 1 ). Of note, patients with low hRAB37 expression were significantly associated with advanced disease (stages III and IV; P =0.005, Pearson χ 2 -test) and with lymph node metastasis ( P =0.013; Fig. 7b and Table 1 ). Importantly, low expression of hRAB37 correlated with worse prognosis in overall survival ( P <0.001, log-rank test; Fig. 7c ) or progression-free survival ( P =0.016; Fig. 7d ). These clinical results confirmed that hRAB37 is a metastasis suppressor with prognostic implication. Figure 7: Low hRAB37 protein coincides with low TIMP1 level and poor survival of lung cancer patients. ( a ) Immunohistochemistry images of hRAB37 and TIMP1 proteins in normal and tumour lung regions of specimen from lung cancer patients. Scale bars, 250 μm. ( b ) Histogram showing frequency of low hRAB37 protein expression in patients with different stages of cancer and lymph node metastasis status (+, preserved; −, low expression). P values determined using Pearson χ 2 -test. ( c , d ) Overall survival ( c ) and progression-free survival curve ( d ) of Kaplan–Meier method indicated that patients with low hRAB37 protein expression had significantly poorer survival than patients with normal expression (+, preserved; −, low expression). P values determined using log-rank test. ( e ) Confocal immunohistochemistry images of hRAB37 (red), TIMP1 (green) and nucleus staining (blue) in tumour specimen from lung cancer patients. Scare bars, 20 μm. Enlarged images are shown for one patient. ( f ) Concordance analysis between hRAB37 and TIMP1 proteins expression (+, preserved; −, low expression) accordingly to the four molecular subtypes (−,−); (+,−); (+,+) and (−,+). hRAB37 expression is shown before the comma followed by TIMP1 expression. The concordant group included patients with hRAB37, TIMP1 (−,−) and patients with hRAB37, TIMP1 (+,+). P values determined using Pearson χ 2 -test. The percentage of cases is indicated on the pie chart. ( g ) Histogram showing frequency of low protein expression of TIMP1 in patients with different stages of cancer and lymph node metastasis status (+, preserved; −, low expression). P values determined using Pearson χ 2 -test. ( h ) Overall survival curve of Kaplan–Meier method indicated that patients with low TIMP1 protein expression had significantly poorer survival than patients with normal expression (+, preserved; −, low expression). P values determined using log-rank test. ( i ) Kaplan–Meier survival curves with respect to hRAB37 or TIMP1 protein expression (+, preserved; −, low expression). P values determined using log-rank test. Full size image Table 1 Alteration of hRAB37 and TIMP1 protein expression levels in relation to clinicopathological parameters in 165 lung cancer patients*. Full size table The relationship between hRAB37 and TIMP1 expression has never been examined in human cancer patients; we therefore performed double fluorescence and confocal immunohistochemistry on lung tumour specimens. Strikingly, confocal immunohistochemistry demonstrated that patients with low hRAB37 showed concordantly reduced TIMP1 ( P <0.0001; Fig. 7e,f and Table 1 ; and Supplementary Fig. 11 ). Patients with low TIMP1 expression were significantly associated with advanced disease (stages III and IV) and with lymph node metastasis ( Fig. 7g and Table 1 ). Indeed, low expression of TIMP1 correlated with poor prognosis in overall survival ( Fig. 7h ). Importantly, patients with low expression of hRAB37 and TIMP1, singly or together, showed significantly worse survival compared with those patients with expression of both proteins ( Fig. 7i ). Altogether, these clinical data demonstrated that low hRAB37 protein coincided with low TIMP1 level in tumour tissues, and reduced expression of both hRAB37 and TIMP1 in surgical specimens are prognostic biomarkers for lung cancer. We conducted an analysis of The Cancer Genome Atlas (TCGA) data set for lung squamous cell carcinoma and lung adenocarcinoma [27] , [28] looking at the mRNA expression levels of hRAB37 and TIMP1 ( Fig. 8a and Supplementary Data 2 ). There was a significant concordance of hRAB37 and TIMP1 expression level in the data set of 450 lung cancer patients ( P <0.001; Fig. 8b and Supplementary Data 3 ). Importantly, patients with lower mRNA level of hRAB37 correlated with advanced tumour stages and had a worse survival ( Fig. 8c,d and Supplementary Data 3 ) than patients with higher level of hRAB37 , indicating that the relevance of our finding was also seen in a large cohort of patients as part of TCGA project. 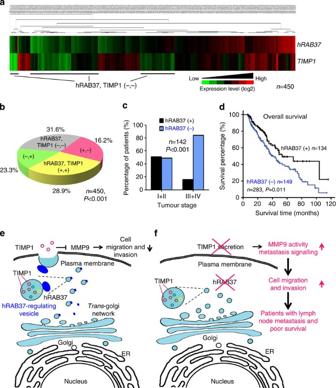Figure 8: LowhRAB37coincides with lowTIMP1level, leading to poor survival of lung cancer patients in the TCGA data set. (a) Expression profiles forhRAB37andTIMP1across 450 human lung tumours in TCGA data set, separated accordingly to the four molecular subtypes (−,−); (+,−); (+,+) and (−,+).hRAB37mRNA expression is shown before the comma followed byTIMP1expression. +, preserved; −, low expression. Mean expression of log2hRAB37andTIMP1was used as the cutoff value. (b) Concordance analysis betweenhRAB37andTIMP1expression (+, preserved; −, low expression). The concordant group included patients withhRAB37,TIMP1(−,−) and patients withhRAB37,TIMP1(+,+).Pvalues determined using Pearsonχ2-test. The percentage of cases is indicated on the pie chart. (c) Overall survival curve of Kaplan–Meier method in patients with preserved and low (< log2 mean)hRAB37mRNA expression (+, preserved; −, low expression).Pvalues determined using log-rank test. (d) Histogram showing frequency of low mRNA expression ofhRAB37in patients with different stages of cancer (+, preserved; −, low expression).Pvalues determined using Pearsonχ2-test. (e,f) Schematic diagram of hRAB37-mediated TIMP1 secretion to inhibit cell migration and invasion. (e) hRAB37, a small GTPase in the exocytotic pathway from the Golgi to the PM, is a migration/invasion suppressor in normal physiological condition. (f) hRAB37-deficient cells reduce TIMP1 secretion into the extracellular compartment, thus resulting in activation of MMPs-mediated motility control signalling. Lung cancer patients with low hRAB37 protein expression coinciding with low TIMP1 expression in their tumours show high lymph node metastasis and poor survival. ER, endoplasmic reticulum. Figure 8: Low hRAB37 coincides with low TIMP1 level, leading to poor survival of lung cancer patients in the TCGA data set. ( a ) Expression profiles for hRAB37 and TIMP1 across 450 human lung tumours in TCGA data set, separated accordingly to the four molecular subtypes (−,−); (+,−); (+,+) and (−,+). hRAB37 mRNA expression is shown before the comma followed by TIMP1 expression. +, preserved; −, low expression. Mean expression of log2 hRAB37 and TIMP1 was used as the cutoff value. ( b ) Concordance analysis between hRAB37 and TIMP1 expression (+, preserved; −, low expression). The concordant group included patients with hRAB37 , TIMP1 (−,−) and patients with hRAB37 , TIMP1 (+,+). P values determined using Pearson χ 2 -test. The percentage of cases is indicated on the pie chart. ( c ) Overall survival curve of Kaplan–Meier method in patients with preserved and low (< log2 mean) hRAB37 mRNA expression (+, preserved; −, low expression). P values determined using log-rank test. ( d ) Histogram showing frequency of low mRNA expression of hRAB37 in patients with different stages of cancer (+, preserved; −, low expression). P values determined using Pearson χ 2 -test. ( e , f ) Schematic diagram of hRAB37-mediated TIMP1 secretion to inhibit cell migration and invasion. ( e ) hRAB37, a small GTPase in the exocytotic pathway from the Golgi to the PM, is a migration/invasion suppressor in normal physiological condition. ( f ) hRAB37-deficient cells reduce TIMP1 secretion into the extracellular compartment, thus resulting in activation of MMPs-mediated motility control signalling. Lung cancer patients with low hRAB37 protein expression coinciding with low TIMP1 expression in their tumours show high lymph node metastasis and poor survival. ER, endoplasmic reticulum. Full size image Here we show that TIMP1 is a novel cargo of hRAB37. We provide compelling evidence from lung cells, animal and clinical studies that hRAB37 is a metastasis suppressor via regulating TIMP1 for exocytosis leading to inactivation of MMP9 signalling with clinical implication of prognosis prediction ( Fig. 8e,f ). Together, our findings that hRAB37 acts as a metastasis suppressor by regulating the exocytotic transport of TIMP1 in a nucleotide-dependent manner to inhibit cancer cell migration and invasion reveal the involvement of a novel component of the vesicular exocytotic machinery in tumour progression. Low or inactive hRAB37 expression promoted metastasis of lung cancer but altered hRAB37 expression had no effect on lung tumour xenograft growth ( Supplementary Fig. 12 ). In the lung-to-lung metastasis animal model, the primary growth judging by the estimated overall tumour sizes of the implanted tumours within the left lateral pleural cavity appeared to be similar among sh-control, sh1 and sh2 groups. Notably, the softer tumours in sh1 and sh2 groups were substantially more dispersed and easily detachable with irregular surfaces compared with the tumours in the control group in which the solid mass was better encapsulated. In line with these observations, the tumours in sh-RAB37 groups showed more parietal and visceral pleura invasion and even invaded the lung parenchyma, consequently leading to higher metastases in the contralateral lungs. Our study demonstrates that hRAB37 is a bona fide metastasis suppressor Rab. According to the multilevel information provided in TCGA, homozygous deletion of hRAB37 has been found in patients with breast invasive carcinoma and ovarian serous cystadenocarcinoma, as well as cell lines from intestine and ovary cancers. Note that G52W and R91W missense mutations, and R93* nonsense mutation were reported for TCGA lung adenocarcinoma as well as uterine corpus endometrioid carcinoma tumours, respectively. In addition, we showed that hRAB37 mRNA was downregulated in some of the liver and colon tumour samples ( Supplementary Fig. 13 ). These findings suggested that hRAB37 may also act a suppressor in liver, colon and other cancers, which warrants further investigations. Most of the previously reported Rab proteins, such as Rab8, Rab11, Rab21, Rab23, Rab25 and Rab27B (refs 3 , 4 , 5 , 6 , 7 , 8 , 9 ), function as metastasis promoters, although Rab25 acts as a tumour growth suppressor in intestinal epithelial cells from the Apc Min/− ; Rab25 −/− mice background [11] . These results indicated that Rab25 is an oncogene-like protein that promotes tumour growth in ovarian and breast cancer models [4] , [5] , but acts as a tumour growth suppressor in intestinal epithelial cells, which raises the question of why the same Rab protein functions differently in different cancers. Such discrepancy was also found for hRAB37 in lung cancer and renal cell carcinoma where KD of hRAB37 reduced cell growth of renal cell carcinoma cell lines [29] . Vesicle isolation assays indicated that TIMP1 was not present in the hRAB37-containing vesicles of renal cell carcinoma cells in which hRAB37 functions as an oncogene ( Supplementary Fig. 14 ). The context-dependent role of Rabs to serve either as an oncoprotein or tumour suppressor may be owing in part to the interaction with different effectors in various tumours [30] . Our proteomics screens and Gene Ontology (GO) analysis revealed that hRAB37 trafficking components were involved in multiple cell biological functions such as cell adhesion, migration, ECM remodelling, actin-mediated cell contraction and cell morphogenesis processes, further supporting the roles of hRAB37 in metastatic control ( Supplementary Fig. 1a ). Moreover, disease biomarker analysis showed that alteration of these putative secreted cargos are mainly involved in tumour progression, including lung cancer ( Supplementary Fig. 1b ). The range of trafficking cargos or effector proteins of hRAB37 involved in the control of metastasis will be further analysed. In addition, whether the function of other secretory Rabs such as Rab3, Rab26 and Rab27A/B are altered in hRAB37-inhibited cells is worthy of further studies. Our immuno-EM observation that dominant-negative T43N-hRAB37 lost membrane binding to the TIMP1-containing vesicles extends the notion that hRAB37 facilitates vesicle docking and fusion but does not affect TIMP1 vesicle formation. Notably, T43N-hRAB37 displayed a perturbed distribution profile with increased perinuclear localization. It raises intriguing questions of how other proteins such as effector and adaptor proteins or other Rabs contribute to regulate TIMP1 sequestration and vesicle formation. Munc13-1 has been shown to function as an effector of mRab37-mediated TNF-α secretion in activated macrophages [16] . Investigations of effectors of hRAB37-mediated trafficking and migration inhibition under stimulated conditions will shed light on the physiological role of hRAB37 (ref. 31 ). Although TIMP1 shows paradoxical effects on tumour growth and metastasis [32] , [33] , and very little is known about its mode of secretion, we demonstrate that hRAB37 directs TIMP1 secretion in a nucleotide-dependent manner to inhibit tumour metastasis attributing to its MMP inhibitor activity. In agreement, TIMP1 inhibits the invasion and metastasis of malignant tumour cells mainly owing to its role as an inhibitor of MMPs [34] , [35] . Of note, our immunohistochemistry in patient specimen and animal xenograft demonstrated that reduced TIMP1 often occurred in tissue specimens with low hRAB37. Reduced TIMP1 expression may result from additional alterations such as promoter hypermethylation of TIMP1 in resected lung tumour [36] . In stratification analyses, low expression of hRAB37 and TIMP1, singly or together, correlated with poor overall survival. From a clinical point of view, it is therefore of particluar interest that low expression of TIMP1 in resected lung tumour tissue could be also an effective prognosis marker. However, other reports indicate that high TIMP1 levels in blood are associated with poor prognosis in some cancers [37] , [38] . A murine model of experimental liver metastasis suggests that the metastasis-mediated by TIMP1 may depend on the specific microenvironmental context [39] . Similarly, stromal caveolin-1, which is transported from the Golgi complex by the exocytotic pathway, also modulates the microenvironment during tumour invasion [40] . The roles of TIMP1 in local and distant extracellular environments are worthy of further interrogations. Our previous DNA methylation and deletion studies have suggested that hRAB37 may be a tumour suppressor, but the mechanism of its anti-metastatic property is not known. The present results identify a novel link that hRAB37 is a metastasis suppressor via regulating TIMP1 for exocytosis to inactive MMP9 invasion signalling. Therapeutic strategies such as DNA demethylation of hRAB37 gene (ref. 14 ) and increased stability of hRAB37 protein [41] could facilitate the development of cancer therapy. Cell culture and transfection reagents Human lung cancer cell lines CL1-0 and CL1-5 were derived from Taiwanese patients with lung adenocarcinoma [42] . A549, H460 and monkey kidney cells COS1 were purchased from the American Type Culture Collection. All cells were maintained in DMEM (Gibco), with 10% fetal bovine serum (Gibco) and 1% penicillin/streptomycin (Gibco), and cultured at 37 °C with 5% CO 2 in air. To generate stable WT, Q89L and T43N cells, cDNAs of hRAB37 were cloned into the pLP’s-Flag vector (Clontech) and transfected into CL1-5 cells by electroporation (Digital Bio Technology, Seoul, Korea). G418 (1,000 μg ml − 1 , Invitrogen) was used to select the stable cells. To KD hRAB37 (L-008933-01-0020) and TIMP1 (L-011792-00-0005), siRNA oligos (Thermo Fisher Scientific Dharmacon RNAi Technologies) were transfected into COS1 or CL1-5 cells at a final concentration of 100 nmol using Lipofectamine 2000 (Invitrogen). To stably KD hRAB37 in the H460 cell line, cells were infected with control and sh-hRAB37 lentiviral particles produced in packaging vector pLKO_TRC005. The viruses were obtained from the RNAi core (Academia Sinica, Taiwan). The KD sequences for hRAB37 sh1; 5′- CCGGAGCTTCCAGATCCGAGACTATCTCGAGATAGTCTCGGATCTGGAAGCTTTTTTG -3′, and for hRAB37 sh2; 5′- CCGGAGCGTCACCCATGCTTATTACCTCGAGGTAATAAGCATGGGTGACGCTTTTTTTG -3′ were used. Cells were selected with puromycin (2.5 μg ml − 1 ) for 1 week after 24 h of infection with control or sh-hRAB37 lentiviral particles with polybrene (4 μg ml − 1 , Sigma-Aldrich). hRAB37 KD efficiency was checked by western blotting. Generation of hRAB37 antibody hRAB37-specific peptide QADEP SFQIR DYVES QKKRS SC (0.1 mg in 200 μl) was injected subcutaneously (s.c.) into the flanks of mice once every 2 weeks. Mice were killed to collect serum containing antibody after 3 months post injection. Western blots were performed to detect the specificity of hRAB37 antibody ( Supplementary Fig. 15 ). The antibody was generated by LTK BioLaboratories, Taiwan. VSVG transport and Tfn recycling assays Cos1 cells were co-transfected with VSVG-ts045-GFP (kindly provided by Dr Jennifer Lippincott-Schwartz at Cell Biology and Metabolism Program, National Institutes of Health, USA), control or hRAB37KD siRNA, and mcherry (to mark the transfected cells) at a ratio of (2.5:5: 1; wt/wt) and were incubated at 40 °C for 6 h post transfection. After 20 h of incubation, cycloheximide (150 ng ml − 1 ) was added to the culture medium and the cells were incubated at 32 °C to allow VSVG transport. Cells were fixed with 4% formaldehyde and stained with 4',6-diamidino-2-phenylindole at various time points. VSVG arrival at the PM was analysed by epifluoresrescence microscopy and the percentage of cells displaying VSVG-tsO45-GFP at the PM was scored in 150 transfected cells in each experiment. For quantifying the release of internalized Tfn, COS1 cells were transfected with control or hRAB37KD siRNA. At 48 h post transfection, cells were serum-starved for 3 h and incubated with AlexaFluor488-conjugated Tfn (Molecular Probes) at 37 °C for 60 min. After three washes with ice-cold PBS containing 0.1% bovine serum albumin (BSA), cells were stripped of surface-bound Tfn with ice-cold acid buffer (150 mM NaCl and 100 mM glycine, pH 3.0). Cells were incubated in medium containing unlabelled holo-Tfn at 37 °C for various time points, washed with PBS and lysed using lysis buffer (0.5% Triton X-100 in PBS). AlexaFluor488-conjugated Tfn was quantified by enzyme-linked immunosorbent assay (ELISA) and normalized with the total protein concentration in cell lysates at each time point compared with time point zero. CM preparation Serum-free CM was prepared from cells (1 × 10 7 ) cultured with 20 ml serum-free medium for 24 h. The cell viability was ascertained using the Trypan blue dye exclusion assay and was >98%. The media were collected following the protocol of Amicon Ultra centrifugal filter units (UFC900396, Millipore) and the Bradford assay (Bio-Rad Laboratories) was used to determine the total protein concentration in the CM samples and cell motility analysis. Proteomics analysis and GO analysis A total of 100 μg of CM was mixed with 4 × SDS sample buffer and 0.5 M DTT and then boiled for 10 min at 95 °C. Samples were run on NuPAGE 4–20% Bis-Tris gradient gels (Invitrogen) in denaturating SDS buffer, then stained using 0.5% Coomassie Brilliant Blue (Bio-Rad Laboratories). The gel pieces corresponding to the differential proteins (control versus WT) were diced into ~1 mm 3 pieces. For in-gel digestion, peptides were extracted twice with 100 μl of 50% acetonitrile in 5% formic acid. The extracted peptides were enriched using OMIX C18 pipet tips (Varian) to remove the effects of any remaining reagents on the iTRAQ labelling [43] . The enriched peptides were then labelled with the isobaric tags for relative and absolute quantification using iTRAQ reagent (Applied Biosystems). Before labelling, iTRAQ-labelled samples were reconstituted and analysed by liquid chromatography-MS/MS. Peptide fragmentation by collision-induced dissociation was performed automatically using the information-dependent acquisition in Analyst QS v1.1 (Applied Biosystems). For identification of proteins, raw MS/MS files were batch-searched against the Swiss-Prot human sequence database (version 20090616; 468851 sequences) using the MASCOT algorithm (v2.1.0, Matrix Science, London, UK). For quantification of proteins, data analysis for the iTRAQ (Isobaric Tags for Relative and Absolute Quantization) experiments was performed with the software Multi-Q [44] . The identified proteins were analysed using the SignalP [45] , SecretomeP [46] and ExoCarta [47] programs to predict the possibility of protein secretion through classic or nonclassic secretion pathways and the presence of transmembrane domains in the protein sequence. The molecular functions of the identified proteins were determined based on a search against the Human Protein Reference Database ( http://www.hprd.org/ ). For pathway analysis, proteins were uploaded and analysed for evidence of an interaction network using MetaCore from GeneGo Inc. ( http://www.genego.com/metacore.php ). The GO analysis was performed by home-made script. In this script, GO terms were assessed by Fisher’s exact test with Benjamini–Hochberg procedure. The enriched GO terms were visualized using Enrichment Map [48] , a Cytoscape plugin. Vesicle isolation and immunoprecipitation Vesicle isolation procedures are modified from Hendrix’s report [9] . In brief, cells (2 × 10 8 ) were sonicated on ice, vesicles were then isolated by centrifugation at low speed (3,000 g for 10 min at 4 °C) and high speed (30,000 g for 60 min at 4 °C) using 40-Ti rotor (Beckman). Supernatant containing vesicles (500 μg) was incubated with anti-Flag antibody to isolate hRAB37-specific vesicles ( Supplementary Table 2 ). Confocal and EM imaging Transfected cells (1 × 10 5 ) were fixed and then incubated with primary and secondary fluorescent antibodies ( Supplementary Table 2 ), and analysed by Olympus FV1000 confocal microscope. For immuno-EM analysis, cells were fixed, sectioned and immersed in H 2 O 2 for 10 min, blocked with 1% BSA for 1 h and then incubated with indicated antibodies and protein A coupled to 10 or 15 nm gold particles ( Supplementary Table 2 ). Sections were post stained with uranyl acetate and lead citrate, and then examined by Hitachi electron microscope (H7650). To measure the co-localization of hRAB37 and TIMP1 in the same vesicles, we obtained >60 immuno-EM images each from control, WT, Q89L and T43N groups. The representative images are shown in Fig. 2c . We then quantified co-localization of both TIMP1 and hRAB37 in the same vesicle of 100 TIMP1-containing vesicles each in control, WT, Q89L and T43N cells. These quantitative procedures were done by two independent immuno-EM experiments, which are shown in Fig. 2d . TIRF imaging CL1-5 cells were seeded on 29-mm glass bottom dish. After 24 h, cells were transiently co-transfected with RFP-hRAB37/GFP-TIMP1 or RFP-vector/GFP-vector for 24 h before image analysis. TIRF system was built on an inverted microscope (Olympus IX81, Japan). The system was equipped with a high-sensitivity EMCCD camera (iXOn3897, Andor Technology) and a UPON × 100 OTIRF objective lens (numerical aperture=1.49; Olympus) to achieve TIRF. GFP and RFP were excited with 491 and 561 nm solid lasers, respectively (100 mW, 10–30% power) and driven by Xcellence software (Olympus imaging software). To capture the hRAB37 trafficking events, images sequences were recorded in stream mode and the frame rate was 30 frames for 1 min. For quantification of vesicle trafficking event, we defined each yellow fluorescence spot as a TIMP1-containing vesicle and trafficking by hRAB37 in cells, and then tracked each yellow vesicle trafficking distance with trackIT software (Olympus). The cutoff length of moving vesicle was 3 μm. The vesicle trafficking event was measured as the ratio of moving yellow vesicles to the total yellow vesicles in cells. For each experimental condition, a total of at least 20 co-localized yellow vesicles per cell were tracked and six cells were scored. Immunoblotting Cells were lysed in 1 × RIPA lysis buffer with a cocktail of antiproteases (Sigma-Aldrich), equal amounts of total cellular extracts were electrophoresed by SDS–PAGE and transferred on to a polyvinylidene difluoride membrane. Primary antibodies used for immunoblotting are list in Supplementary Table 2 . Full-length images of immunoblots are shown in Supplementary Fig. 16 . Enzyme-linked immunosorbent assay The TIMP1 (Invitrogen) and TNF-α (R&D Systems) ELISA kits were used to detect TIMP1 and TNF-α concentration in CM according to the manufacturer’s protocol. The standards and CM samples were added into 96-well plate that contains antibody. The biotin conjugate solution was added into the wells and incubated at room temperature for 2 h. After incubation, wells were washed with wash buffer and incubated with streptavidin-horseradish peroxidase working solution. Stabilized chromogen and stop solution were then added. The absorbance is measured at 450 nm using an ELISA plate reader. Gelatin-zymography assay CM were collected and analysed by gelatin-zymography in 0.1% gelatin-8% acrylamide gels. After electrophoresis, gel was washed with 2.5% Triton X-100 to remove SDS and renature MMP9. Gel was then incubated overnight in the developing buffer to induce gelatin lysis by renatured MMP9 and stained with 0.5% Coomassie blue G for 1 h. The proteolytic activities were identified as clear bands. Migration and invasion assays For transwell migration assay, cells (1 × 10 5 ) were placed in the upper chamber of transwell (Falcon) with serum-free medium. For transwell invasion assay, the transwell membranes were pre-coated with Matrigel (2.5 mg ml − 1 , Sigma-Aldrich). Medium containing 10% fetal bovine serum was added to the lower chamber as chemoattractants and cells were incubated at 37 °C for 16 h. Cells attached to the reverse side of the membrane were stained with crystal violet, and 10 randomly selected fields were counted under inverted microscope (Nikon TS100) for each experiment. Experimental metastasis assays in vivo The use and care of the BALB/c nude mice were approved by the Institutional Animal Care and Use Committee of National Cheng Kung University. Three groups of animals were used; the first group included control, WT, Q89L and T43N stable expression CL1-5 cells. In the second group, WT-Con, WT-TIMP1KD and WT-TIMP1KD+TIMP1 CL1-5 cells were used. In the third group, T43N stable expression CL1-5 cells treated with (+TIMP1) or without (T43N) recombinant TIMP1 protein (410-01, Peprotech) for 24 h. For these three groups, cells were resuspended in serum-free medium (2 × 10 6 cells per 200 μl) and intravenously injected via the tail vein into BALB/c nude mice. Mice were killed after 6–8 weeks and lung tissues were resected, fixed and embedded in paraffin for histological H&E and immunohistochemistry staining. Lung-to-lung metastasis assay in vivo Six-week-old male BALB/c nude mice were purchased from BioLASCO (Taipei, Taiwan) and acclimated for 2 weeks in the animal facilities at the National Health Research Institutes (NHRI), Taiwan. All animal treatments and experimental protocols for this study were reviewed and approved by the Institutional Animal Care and Use Committee at NHRI. Mice were divided into eight mice per group. Stable hRAB37 KD (sh1 and sh2) and sh-control H460 cells were used. A total of 5 × 10 4 cells were suspended in 100 μl Matrigel (Becton Dickinson) in PBS. Mice anaesthetized with isoflurane were placed in the right lateral decubitus position. Tuberculin syringes (1 ml) with 26-gauge hypodermic needles were used to inject the cell inoculum percutaneously into the left lateral thorax, at the lateral dorsal axillary line, 1.5 cm above the lower rib line just below the inferior border of the scapula. The needle was quickly advanced 5–7 mm into the thorax and was quickly removed after the injection of cell suspension. After tumour injection, the mouse was turned to the left lateral decubitus position. Animals were observed for 45–60 min until fully recovered. Four weeks after cell inoculum, animals were killed. The solitary lesions located in the injected left lateral lung and within the pleural thoraxes were removed. The contralateral lungs were isolated and prepared for pathological examination. Lung tissues were fixed with 10% neutral buffered formalin for 48 h before tissue processing, which included dehydration, and embedding in paraffin. H&E stain was used for general histopathological examinations. The outward appearance of the lungs and the solitary nodules were recorded. Tumour growth assay in vivo Six-week-old BALB/c nude mice, approved by the Institutional Animal Care and Use Committee of National Cheng Kung University, were s.c. inoculated with vector control and hRAB37-WT stable expression CL1-5 cells (1 × 10 7 cells per 100 μl) and allowed to grow for 21 days. The animals were maintained under sterile conditions in laminar flow rooms and provided with sterilized food and water. After 3 weeks, the mice were killed and the tumour xenografts were removed, photographed and weighed. Patient samples and clinical information A total of 165 lung cancer patients were recruited from Taipei Veterans General Hospital between 1999 and 2010 after obtaining appropriate institutional review board permission and written informed consent from patients. Paraffin blocks of tumours were collected. The detailed clinicopathological characteristics of the enrolled patients are listed in Supplementary Table 1 . Immunohistochemistry and fluorescence immunohistochemistry Immunohistochemistry was performed to detect protein expression of hRAB37 and TIMP1 in tumour sections from lung cancer patients. Staining for expression region was scored as follows: absent (0–25%), decrease (25–50%) and preserve (>50%), while absent and decrease was defined as protein low expression. The surrounding normal tissue served as an internal positive control for each slide. For fluorescence immunohistochemistry and confocal microscopy of hRAB37 and TIMP1 localization, primary antibody followed by incubation with the fluorescent secondary antibodies and 4',6-diamidino-2-phenylindole ( Supplementary Table 2 ) for 1 h, after which images were obtained with confocal microscope. mRNA expression analysis For hRAB37 mRNA expression assay, a semi-quantitative reverse transcription PCR assay using the GAPDH gene as an internal control to indicate the amount of RNA in each reaction was performed. The primer nucleotide sequences are as follows: for hRAB37 gene, sense, 5′- ACGGGCAAGGTGATGCTTCTGG -3′, antisense, 5′- CATCTCTGTAATAAGCATGGGTGACGCT -3′; for the GAPDH gene, sense, 5′- AATCCCATCACCATCTTCCA -3′, antisense, 5′- CCTGCTTCACCACCTTCTTG -3′. PCR was performed for 34 cycles with annealing temperature of 68 °C using cDNA synthesized from total RNA. TCGA analysis The analysis of the TCGA data set for lung cancer was conducted through the cBio Cancer Genomics Portal [28] based on the 24 October, 2012 Broad Firehose run of TCGA data. Expression and survival data of patients are presented in Supplementary Data 2 and 3 . The data were normalized and log2 was transformed. Statistical analysis Pearson χ 2 -test was used to compare the altered frequency of hRAB37 and TIMP1 between lung cancer patients with different clinicopathological parameters. Overall survival and disease-free survival curves were calculated according to the Kaplan–Meier method, and comparison was performed using the log-rank test. Two-tailed Student’s t -test was used in cell and animal studies. Three independent experiments for cell studies and eight mice per group for animal studies were analysed unless indicated otherwise. Data represent mean+s.e.m. P <0.05 was considered to be statistically significant. How to cite this article: Tsai, C.-H. et al . Small GTPase Rab37 targets tissue inhibitor of metalloproteinase 1 for exocytosis and thus suppresses tumour metastasis. Nat. Commun. 5:4804 doi: 10.1038/ncomms5804 (2014).